Crystal structure of the yeast TSC1 core domain and implications for tuberous sclerosis pathological mutations Tuberous sclerosis complex is a disease caused by mutations in two tumor-suppressor genes, TSC1 and TSC2. The TSC1 protein, also known as hamartin, has a critical role in controlling mTOR signalling. TSC1 does not bear apparent sequence homology with other proteins. Here we show that the N-terminal half of yeast TSC1 forms a protease-resistant domain, which is evolutionarily conserved. The crystal structure of this yeast TSC1 core domain shows that it contains a pseudo-HEAT repeat fold with its C-terminal end capped by a helical subdomain. This allows us to model the three-dimensional structure of the human TSC1 N-terminal domain (TSC1-NTD), which anchors essentially all pathogenic TSC1 missense mutations found in tuberous sclerosis patients. Interestingly, most pathogenic mutations map inside of the folded TSC1-NTD structure, whereas most non-pathogenic variants are on the structural surface. This indicates that the disruption of the TSC1-NTD globular structure is a major cause of tuberous sclerosis. Tuberous sclerosis or tuberous sclerosis complex (TSC) is an autosomal-dominant disease characterized by the development of tumor-like growths, named hamartomas, in the kidneys, heart, skin and brain. The major features of tuberous sclerosis include dermatological manifestations, renal angiomyolipomas, neurological manifestations, pulmonary lymphangiomyomatosis and malignancy in some cases [1] , [2] . Tuberous sclerosis is caused by the mutation of one of two tumor-suppressor genes, TSC1 and TSC2 , which encode TSC1 (hamartin) and TSC2 (tuberin) proteins, respectively [3] . TSC1 and TSC2 homologues have been identified in a range of eukaryotes, including S. pombe . TSC1 and TSC2 proteins form a complex and regulate cell physiology, growth and proliferation. Although other downstream pathways are also likely, the TSC1–TSC2 complex suppresses cell growth largely by inhibiting small G-protein Rheb, a crucial activator of the mTORC1 pathway [2] , [4] , [5] , [6] , [7] , [8] , [9] , [10] , [11] , [12] . Phosphorylation of TSC1 and TSC2 by a number of upstream kinases (for example, AMPK, Akt and GSK3) and binding of their protein partners, including TBC1D7, has an important role in controlling the TSC1–TSC2 complex formation and the output to the mTORC1 pathway [2] , [4] , [5] , [6] , [7] , [8] , [9] , [10] , [11] , [12] , [13] , [14] . In the TSC1–TSC2 complex, TSC1 is believed to enhance TSC2 function by activating the TSC2 GAP activity, stabilizing the TSC2 protein in the cell and/or correct intracellular localization of the TSC1–TSC2 complex [15] , [16] , [17] , [18] , [19] , [20] , [21] . TSC1 protein has many binding partners in addition to TSC2, and is essential for mouse embryonic development [22] , [23] , [24] . Recently, it has been shown that TSC1 has critical roles in neurodevelopment and neurological diseases, immune diseases, diabetes, autophagy and DNA repair [25] , [26] , [27] , [28] . Similar to the signalling mechanism in mammalian cells, the TSC1–TSC2 complex in S. pombe also regulates the TOR kinase activity, and has a role in amino-acid uptake from the environment and amino-acid homeostasis [29] , [30] , [31] . Human TSC1 shares sequence homology with the yeast TSC1 [29] . The most conserved region is the hTSC1 region spanning the N-terminal ~265 residues, which anchors a majority of disease-associated TSC1 mutations identified. Some of these mutations are missense mutations, but only a fraction of these TSC-associated missense mutations are actually disease causing (pathogenic) [32] , [33] , [34] . All pathogenic TSC mutations result in a loss of TSC1 protein in the cell and increased TORC1 signalling [32] . Previous work also showed that all these pathogenic TSC1 missense mutations are located in the N-terminal domain of TSC1 (TSC1-NTD), in particular between amino acids 50 to 224 [32] , [33] , [34] . Given the large size of the TSC1 protein, it is quite striking that this short TSC1 region accounts for all known pathogenic TSC1 mutations. TSC1-NTD is conserved among all TSC1 proteins, including that from S. pombe , and may contribute to its interactions with TSC1 partners, in addition to TSC1 stability [22] , [35] . Except for the TSC2 GAP domain that shares sequence homology with the Rap family of small G-protein, TSC1 and TSC2 have no apparent sequence homology with other proteins. Despite tremendous efforts in many structural labs, because of the difficult biochemical properties of TSC1 and TSC2 proteins, no crystal or NMR structure has been reported for any part of the TSC1 and TSC2 proteins. There is no doubt that three-dimensional (3D) structures of TSC1 and TSC2 will be crucial for understanding the molecular mechanisms of TSC and for developing novel approaches for TSC treatment. Our knowledge of TSC has been hindered by a lack of 3D structure of TSC1/2 proteins. Here we show that yeast TSC1 contains a protease-resistant core domain, and through the determination of crystal structure, we reveal the first 3D structure of TSC1. This structure also provides key insights into the molecular mechanism of TSC1 pathogenic mutations. Yeast TSC1 contains a protease-resistant core domain TSC1 of S. pombe (yTSC1) contains 899 residues with a molecular weight of 103 kDa. It is predicted to contain a N-terminal-folded domain and a C-terminal coiled-coil region (residues 540–847; Fig. 1a , Supplementary Fig. S1 ). Full-length yTSC1 was overexpressed in E. coli and purified by a combination of affinity, ion-exchange and size-exclusion chromatography (SEC). SEC analysis indicated that the full-length yTSC1 appears predominantly as a large oligomer with an apparent molecular weight of ~900 kDa ( Fig. 1b ). 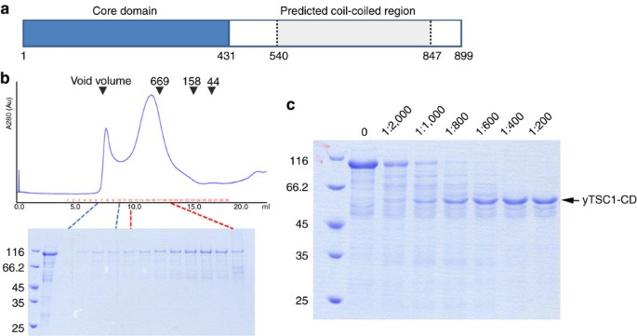Figure 1:Structural characterization of the TSC1 fromS. pombe(yTSC1). (a) Domain structure of yTSC1 is shown. Yeast TSC1 contains the N-terminal core domain (blue) and the predicted C-terminal coiled-coil region (cyan). (b) SEC of yTSC1 demonstrates a stable large yTSC1 oligomer. Full-length yTSC1 (with a nominal MW of ~100 kDa) was loaded to a Superose 6 10/300 GL column, and fractions from the void volume and the main peak were detected by SDS–PAGE. The numbers on top of the chromatograph are positions of standard molecular weight markers (in kilodaltons). (c) Limited proteolysis of yTSC1 reveals that the N-terminal half of yTSC1 forms the protease-resistant core domain of yTSC1. The marked ratios are the trypsin:yTSC1 molecular ratios used in limited proteolysis. Both SDS–PAGE inb,care stained with Coomassie Brilliant Blue. Figure 1: Structural characterization of the TSC1 from S. pombe (yTSC1). ( a ) Domain structure of yTSC1 is shown. Yeast TSC1 contains the N-terminal core domain (blue) and the predicted C-terminal coiled-coil region (cyan). ( b ) SEC of yTSC1 demonstrates a stable large yTSC1 oligomer. Full-length yTSC1 (with a nominal MW of ~100 kDa) was loaded to a Superose 6 10/300 GL column, and fractions from the void volume and the main peak were detected by SDS–PAGE. The numbers on top of the chromatograph are positions of standard molecular weight markers (in kilodaltons). ( c ) Limited proteolysis of yTSC1 reveals that the N-terminal half of yTSC1 forms the protease-resistant core domain of yTSC1. The marked ratios are the trypsin:yTSC1 molecular ratios used in limited proteolysis. Both SDS–PAGE in b , c are stained with Coomassie Brilliant Blue. Full size image Limited proteolysis of yTSC1 showed that the N-terminal 431 residues are resistant to proteases, whereas the C-terminal half, including the predicted coiled-coil domain, is sensitive to proteolysis ( Fig. 1c ). This indicates that yTSC1 contains a protease-resistant core domain (yTSC1-CD). Purified yTSC1-CD exists in solution predominantly in dimeric form, as indicated by SEC analysis ( Supplementary Fig. S2 ). Crystal structure of the yTSC1 core domain The yTSC1 core domain was crystallized under different conditions in two different space groups (P2 1 2 1 2 for the form 1 and P2 1 for the form 2; Supplementary Table S1 ). Crystals of these two forms diffracted to 2.9 and 3.3 Å resolutions, respectively ( Fig. 2a , Supplementary Table S1 ). Crystal structure for the form 1 was determined using the selenium-methionine single-anomalous-dispersion method, whereas the form 2 structure was solved with molecular replacement using the structural model derived from the form 1 crystal. In the form 1 crystal structure, there are ten yTSC1-CD molecules in the asymmetric unit, with two pentamers facing each other (‘face-to-face’, Fig. 2b ). In the crystal form 2, there are two decamers, almost identical to the decamer structure in form 1 crystal, in each asymmetric unit ( Supplementary Fig. S3 ). In the decameric structure, all C-termini of the 10 yTSC1(1–431) subunits, as well as a ~20 residue missing loop in each yTSC1-CD structure, are located in the mid-level inside the tunnel ( Fig. 2b ). Whether this decameric oligomer structure is physiologically relevant in the context of full-length protein remains a question (Discussion). As yTSC1(1–431) exists in solution predominantly in dimeric state when the protein concentration is in or below the low μM range, we will mainly focus our discussion on the structure of yTSC1(1–431) dimer. 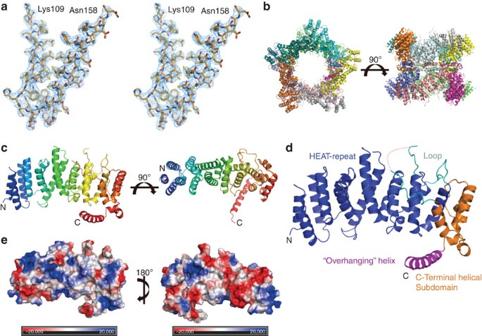Figure 2: Crystal structure of the core domain of yTSC1. (a) Stereo view of a typical area of electron density map. In the crystal form 1 (P21212), yTSC1 residues from 109 to 158 were displayed with electron density calculated using 2Fo-Fc coefficients and contoured at 1.2 σ as a blue mesh. (b) Decameric structure of the yTSC1 core domain in the P21212 crystal lattice. Ten yTSC1-CD subunits in different colours form a two-layer pentagonal ring with a hollow channel in the centre. In the second crystal form (in space group P21), there are two identical decamers in the asymmetric unit (Supplementary Fig. S3). (c) Two orthogonal views of the yTSC1-CD monomer, with the protein coloured in gradient (N- to C-termini, blue to red). (d) Different regions of yTSC1-CD are shown here in different colours. The HEAT-repeat, the long loop, the C-terminal helical subdomain and the C-terminal ‘overhanging’ helix are showed in blue, cyan, orange and magentas, respectively. The two ends of the disordered long loop were connected by a dashed red line. (e) Electrostatic surface presentation of yTSC1-CD is calculated with the APBS plugin in Pymol. Blue and red represent positive and negative potentials at the 20 k Te−1and −20 k Te−1scales. Figure 2: Crystal structure of the core domain of yTSC1. ( a ) Stereo view of a typical area of electron density map. In the crystal form 1 (P2 1 2 1 2), yTSC1 residues from 109 to 158 were displayed with electron density calculated using 2Fo-Fc coefficients and contoured at 1.2 σ as a blue mesh. ( b ) Decameric structure of the yTSC1 core domain in the P2 1 2 1 2 crystal lattice. Ten yTSC1-CD subunits in different colours form a two-layer pentagonal ring with a hollow channel in the centre. In the second crystal form (in space group P2 1 ), there are two identical decamers in the asymmetric unit ( Supplementary Fig. S3 ). ( c ) Two orthogonal views of the yTSC1-CD monomer, with the protein coloured in gradient (N- to C-termini, blue to red). ( d ) Different regions of yTSC1-CD are shown here in different colours. The HEAT-repeat, the long loop, the C-terminal helical subdomain and the C-terminal ‘overhanging’ helix are showed in blue, cyan, orange and magentas, respectively. The two ends of the disordered long loop were connected by a dashed red line. ( e ) Electrostatic surface presentation of yTSC1-CD is calculated with the APBS plugin in Pymol. Blue and red represent positive and negative potentials at the 20 k Te −1 and −20 k Te −1 scales. Full size image In each yTSC1(1–431) subunit, there is a globularly folded domain, which is composed of 20 helices and an additional helix that points out of the folded domain ( Fig. 2a ). Within the folded domain, the first 14 helices forms a pseudo-HEAT-repeat structure (residues 1–281), followed by a long-loop (residues 281–338), and a helical subdomain capping the C-terminal end of the pseudo-HEAT repeat ( Fig. 2b ). The long loop is not conserved among TSC1 proteins and part of this loop is structurally flexible and not observed in our electron density map ( Fig. 2c and Supplementary Figs S4 and S5 ), whereas the C-terminal helical subdomain is responsible for the dimerization of yTSC1-CD. The free ‘overhanging’ helix (H21, residues 412–430) is involved in the formation of potential decamer structure by mediating the ‘face-to-face’ stacking of the two pentamer rings ( Fig. 2b ). A Dali search showed that the closest structures of yTSC1-CD are the PP2A B56 regulatory subunit, the CAND structure and the tRNA export factor (Xpot), all of which contain a similar HEAT repeat or pseudo-HEAT repeat structures ( Supplementary Table S2 ). We examined several potential dimeric interfaces within the decamer. Using SEC assay with purified recombinant proteins, we found that while yTSC1(1–431) forms a stable dimer, yTSC1(1–392) that does not contain the H19-H21 segment exists mainly as a monomer. In contrast, yTSC1(1–409) with removal of just H21 still exists mainly as a dimer ( Fig. 3a ). This leads to just one possibility for the dimer interface that involves the H16, H18 and H19, which mediates the ‘end-to-end’ dimerization of the yTSC1-CD helical domain ( Fig. 3c ). Indeed, missense mutations of two key residues involved in this symmetric yTSC1-CD interface (F398A, L399A) completely abolished the dimerization of yTSC1-CD ( Fig. 3b ). This demonstrates that the interface shown in Fig. 3d is responsible for stable yTSC1-CD dimerization in solution. 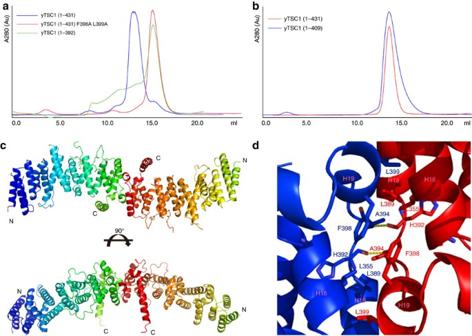Figure 3: Dimeric structure of the yTSC1 core domain. (a) The analytical SEC analyses of yTSC1(1–392) and the yTSC1-CD double mutant (F398A, L399A) were performed with Superdex 200 Hiload 10/300 GL. (b) Comparative SEC analysis of yTSC1(1–431) and yTSC1(1–410) was done using Superdex 200 Hiload 10/300 GL. (c) Overall structure of the yTSC1 dimer (coloured in gradient). The dimer interface is formed by the two pseudo-symmetric C-terminal helical subdomains (H16, H18 and H19). (d) The details of the yTSC1 homodimer interface are shown here. Two yTSC1 molecules are coloured in blue and red, respectively. The residues on the dimer interface are highlighted in stick model. The helices involved in dimerization are labelled in pink. Two mainchain–mainchain hydrogen bonds between His392 and Ala394 are labelled in yellow dash lines. Figure 3: Dimeric structure of the yTSC1 core domain. ( a ) The analytical SEC analyses of yTSC1(1–392) and the yTSC1-CD double mutant (F398A, L399A) were performed with Superdex 200 Hiload 10/300 GL. ( b ) Comparative SEC analysis of yTSC1(1–431) and yTSC1(1–410) was done using Superdex 200 Hiload 10/300 GL. ( c ) Overall structure of the yTSC1 dimer (coloured in gradient). The dimer interface is formed by the two pseudo-symmetric C-terminal helical subdomains (H16, H18 and H19). ( d ) The details of the yTSC1 homodimer interface are shown here. Two yTSC1 molecules are coloured in blue and red, respectively. The residues on the dimer interface are highlighted in stick model. The helices involved in dimerization are labelled in pink. Two mainchain–mainchain hydrogen bonds between His392 and Ala394 are labelled in yellow dash lines. Full size image Structural modelling of human TSC1 N-terminal domain The human TSC1 protein (hamartin) contains 1,164 residues. Other than the predicted coiled-coil region (residues 721–997) and the N-terminal domain (residues 1–270, hTSC1-NTD), other regions of hamartin are predicted to be disordered intrinsically, including the region covering residues 302–420, which is important for TSC2 (tuberin) binding [5] . Sequence alignment of yeast and human TSC1 proteins demonstrated that hTSC1-NTD is homologous to the yTSC1 core domain ( Fig. 4a ). Specifically, the shorter hTSC1-NTD contains neither the region corresponding to the first 133 residues of yTSC1-CD nor the long-loop between yTSC1 H14 and H15. Excluding these two yTSC1 regions, yTSC1-CD and hTSC1-NTD share 20% identity and 58% homology. A homology-based model for hTSC1-NTD is thus built using MODELLER [36] , [37] . In this model, hTSC1-NTD has a shorter HEAT-repeat domain (without the first six helices in yTSC1) and does not contain the long flexible loop that is unique to yTSC1. Otherwise hTSC1-NTD shares very similar fold with yTSC1-CD ( Fig. 4b ). 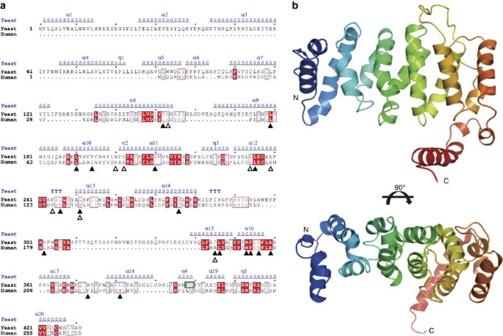Figure 4: A structural model of the N-terminal domain of human TSC1. (a) Sequence alignment of yTSC1-CD with hTSC1-NTD was performed with EBI ClustalW2, thereafter the result was modified by ESPript. Residues with pathogenic mutations and non-pathogenic variants are labelled with solid and empty triangle, respectively. Residues with both solid and empty triangles refer to different missense mutations in the same position. Two key residues (F398, L399) involved in yTSC1-CD dimerization are bracketed. (b) The 3D structure model of hTSC1-NTD is shown in two orthogonal orientations. Figure 4: A structural model of the N-terminal domain of human TSC1. ( a ) Sequence alignment of yTSC1-CD with hTSC1-NTD was performed with EBI ClustalW2, thereafter the result was modified by ESPript. Residues with pathogenic mutations and non-pathogenic variants are labelled with solid and empty triangle, respectively. Residues with both solid and empty triangles refer to different missense mutations in the same position. Two key residues (F398, L399) involved in yTSC1-CD dimerization are bracketed. ( b ) The 3D structure model of hTSC1-NTD is shown in two orthogonal orientations. Full size image To understand the oligomeric state of hTSC1-NTD, we performed SEC analysis, which demonstrated that hTSC1-NTD is mainly monomeric in solution but also contains large oligomeric species ( Supplementary Fig. S6 ). This is consistent with the sequence alignment that shows a lack of sequence conservation of residues in the yTSC1-CD dimerization interface. Thus, we will focus on the hTSC1-NTD monomer for interpreting TSC1 pathogenic mutants. Mapping of TSC1 pathogenic mutations to the TSC1 structure A majority of TSC-associated human TSC1 variants have been mapped to hTSC1-NTD, with some of them being pathogenic and others neutral or non-pathogenic [32] , [33] , [34] . By mapping these missense variants to the hTSC1-NTD model, it is clear that most of the pathogenic mutations are located inside of the hydrophobic cores of TSC1-NTD and would disrupt the folding of hTSC1-NTD ( Fig. 5a ). Some of these mutations, such as L61R, I76N, L93R, G132D, F158S, L191 H/R, F216S and M224R, change the hydrophobic residues into hydrophilic residues and thus are expected to disrupt the structure. A few others, such as V133F, would also destabilize the structure because the hydrophobic core cannot accommodate a much larger side chain. Interestingly, many missense mutations, including L50P, L61P, L72P, L117P, L180P, L191P and R204P, are replacements of amino acids in helices with a proline, which are expected to disrupt the helical secondary structure and lead to misfolding of TSC1-NTD. In addition, there are also some local deletion/insertion mutations, such as N198F199delinsI, that can also disrupt the hydrophobic core and thus destabilize TSC1. 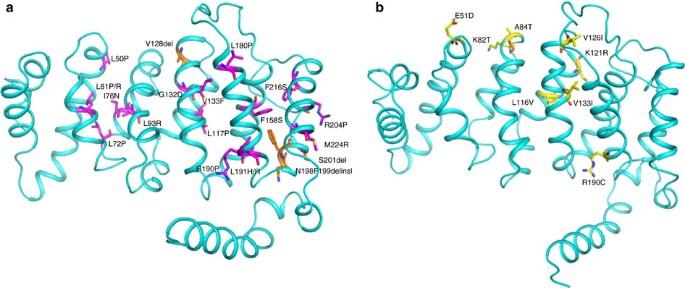Figure 5: Structural basis of the TSC1 pathogenic mutations. (a) Locations of pathogenic TSC1 mutations in the hTSC1-NTD structure model. These mutations include L50P, L61P/R, L72P, I76N, L93R, L117P, G132D, V133F, F158S, L180P, R190P, L191 H/R, R204P, F216S, M224R, V128del, N198F199delinsI and S201del. (b) Locations of non-pathogenic TSC1 mutations in the hTSC1-NTD structure model. These mutations are E51D, K82T, A84T, L116V, K121R, V126I, V133I and R190C. Figure 5: Structural basis of the TSC1 pathogenic mutations. ( a ) Locations of pathogenic TSC1 mutations in the hTSC1-NTD structure model. These mutations include L50P, L61P/R, L72P, I76N, L93R, L117P, G132D, V133F, F158S, L180P, R190P, L191 H/R, R204P, F216S, M224R, V128del, N198F199delinsI and S201del. ( b ) Locations of non-pathogenic TSC1 mutations in the hTSC1-NTD structure model. These mutations are E51D, K82T, A84T, L116V, K121R, V126I, V133I and R190C. Full size image In contrast, almost all non-pathogenic variants of TSC1 are mapped to the surface of hTSC1-NTD model and are not expected to lead to major conformational change ( Fig. 5b ). At least one non-pathogenic variant, that is, L116V, is located inside the structure, which is not expected to disrupt the folded structure due to similar hydrophobic side chains. Overall, our structure model is in excellent agreement with pathogenic properties of TSC1 mutations. Therefore, we conclude that the N-terminal 265 residues of TSC1 forms a globularly folded domain and all pathogenic TSC1 mutations cause tuberous sclerosis by disrupting the folding of this domain. Recent works have demonstrated that TSC1, TSC2 and the TSC1–TSC2 complex are central factors in the mTOR pathway, by integrating extracellular (hormonal) and intracellular (nutritional, cell-cycle and so on) signals to regulate cell physiology, growth and proliferation [2] , [4] , [5] , [6] , [7] , [8] . TSC1 and TSC2 mutations are responsible for tuberous sclerosis and are associated with other diseases including pulmonary lymphangioleiomyomatosis [23] . 3D structures of TSC1, TSC2 and their complex are crucial for understanding their normal function and regulation and the pathogenic mechanism of their mutations. Furthermore, structural studies will be also crucial for developing novel therapeutics for the treatment of TSC and lymphangioleiomyomatosis. Yeast TSC1 contains 899 residues. Other than the region 422–560 predicted to be important for TSC2 binding (based on its weak homology to the hTSC1 302–420) and a predicted coiled-coil region, the domain structure reflecting its 3D structure was essentially unknown. Our limited proteolysis analysis showed that, while the N-terminal half of yTSC1 is resistant to proteolysis, the C-terminal half is sensitive to proteolysis and may not contain any globularly folded domain. Furthermore, our crystal structure shows that the N-terminal core domain is all helical and contains a pseudo-HEAT repeat structure. This will facilitate with the mapping of mutant position, phosphorylation sites and binding surfaces for yTSC1 binding partners. Interestingly, we observed in our crystal lattice decameric ring-like structure consisting two stacked-pentamers. Although the yTSC1-CD structure exists in solution mainly as a dimer, this ring structure may still be physiologically relevant in the context of full-length protein, which forms mainly a large stable oligomer, with a size roughly corresponding to the yTSC1 decamer ( Fig. 1b ). In addition, the same decameric ring was observed in two different crystal forms grown from distinct conditions ( Fig. 2b and Supplementary Fig. S3 ), suggesting that this oligomeric structure of yTSC1-CD is favored at high protein concentrations. The presence of the C-terminal coiled-coil region promotes the oligomerization of yTSC1, which may be sufficient for this concentration effect. Future work will be needed to characterize if the decameric structure can form under certain scenario in the cell. The most conserved region among TSC1 proteins is the N-terminal domain [29] . This is is also the region accounting for all pathogenic TSC1 mutations. It is quite striking that the yeast TSC1 core domain mapped by our limited proteolysis matches perfectly to the hTSC1-NTD. Mapping of TSC1 missense mutations allowed us to conclude that most, if not all, pathogenic TSC1 mutations cause TSC through the disruption of the folded TSC N-terminal domain. From all these results, it is clear that TSC1-NTD folding is crucial for appropriate functioning of TSC1–TSC2. Previously, it has been shown that the hTSC1-NTD is crucial for TSC1 stability in the cell and contributes to TSC2 binding [35] . How does TSC1-NTD stabilize TSC1 and/or TSC2? Protein folding propensity predictions suggest that the N-terminal domain and possibly the coiled-coil domain of hTSC1 are folded ( Supplementary Fig. S7 ). Although hTSC1-NTD is mainly monomeric, all tested hTSC1 fragments containing the coiled-coil domain have strong tendency of aggregation [35] . There are a number of possibilities for explaining the role of TSC1-NTD in TSC1 stability. It may have a role in TSC1 localization, in particular to the cell membrane [38] . In this regard, it is interesting to note that a transmembrane helix was previously predicted. Our structure does not support the existence of such a transmembrane helix but does not exclude the possibility that the TSC1-NTD directly bind to membrane or to a membrane-attached protein. Indeed, one surface of the predicted human TSC1-NTD structure is flat and positively charged, which are typical structural features for membrane-binding surfaces of proteins ( Fig. 6 ). Alternatively, TSC1-NTD may shield the TSC1 structure components needed for TSC1 turnover for protein degradation system. In this regard, it should be noted that TSC1-NTD is required for TSC1 oligomerization and aggregation [35] , which may be important for this potential shielding effect. In summary, we present the first structure of TSC1, which sheds light to the TSC pathological mechanisms and will serve as a foundation for understanding TSC1 function and regulation. 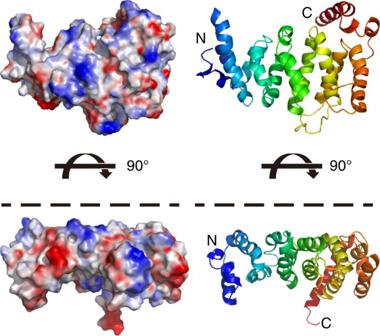Figure 6: A speculated membrane-binding surface of human TSC1-NTD. Two orthogonal views of hTSC1-NTD are shown in top and bottom panels, respectively. Corresponding electrostatic surfaces and cartoon views are shown in left and right, respectively. The flat and positively charged top surface of the upper orientation is predicted to have a role in membrane binding. The dash lines in the bottom panels represent the membrane surface. Figure 6: A speculated membrane-binding surface of human TSC1-NTD. Two orthogonal views of hTSC1-NTD are shown in top and bottom panels, respectively. Corresponding electrostatic surfaces and cartoon views are shown in left and right, respectively. The flat and positively charged top surface of the upper orientation is predicted to have a role in membrane binding. The dash lines in the bottom panels represent the membrane surface. Full size image Protein expression and purification DNA sequences expressing full-length and residues 1 to 431 of TSC1 from Schizosaccharomyces pombe were inserted into a self-made vector named pAL, and then the plasmid was transformed into expression strain BL21(DE3) of Escherichia coli . selenomethionine substituted yTSC1 with N-terminal poly-6His tag was expressed using autoinduction method. Cell pellets were harvested at 4 °C and then resuspended by the lysis buffer. Thereafter, cells were disrupted by sonication following high-speed centrifugation at 15,000 r.p.m. After released to the supernatant, proteins were purified by nickel affinity column, followed by mono Q. TSC1 fractions from mono Q were concentrated and further purified by a Superdex 200 Hiload 16/60 column. Mutant plasmids of yTSC1(1–431) were constructed with the Stratagene Quickchange Kit. DNA sequences encoding residues 1 to 266 of TSC1 from Homo sapiens was also inserted into the vector pAL. Purification of mutants and the homologue of yTSC1(1–431) is the same as the one described above except that the step of mono Q was skipped. yTSC1-CD crystallization and structure determination After purification, yTSC1(1–431) was concentrated to 10 mg ml −1 , and then set for crystal screen using sitting-drop method at room temperature. After initial hit was found, hanging drop vapour diffusion method was employed to optimize crystals. At last, the crystal forms 1 and 2 of yTSC1(1–431) were obtained from 75 mM sodium citrate pH 5.6, 25 mM HEPES pH 7.5, 500 mM NaCl, 1.5% PEI, 6.25% 2-propanol and from 60 mM imidazole pH 7.0, 40 mM CHES pH 9.5, 120 mM NH 4 citrate pH 7.0, 400 mM sodium citrate, 12% PEG MME 2000, respectively. The 2.9 Å resolution SAD data set was collected at BL 8.2.1 and BL 8.2.2 beamlines of the Advanced Light Source in Berkeley at 0.9792 Å. The data set was processed with HKL2000 [39] . The crystal belongs to P2 1 2 1 2 space group and there are 10 molecules in one asymmetric unit. The Se sites were searched by AutoSol in PHENIX [40] , and autobuilding was done with ARP/wARP in CCP4 suite [41] . Model building was performed in COOT [42] and iterative cycles of model building was fulfilled by Refmac5 in CCP4 [41] and PHENIX [40] . Noncrystallographic symmetry restrains were applied to improve the electron density map. The electrostatic potential surfaces shown were generated by the APBS tool in Pymol [43] . Limited proteolysis FL-His-yTSC1 was mixed with trypsin at different molar ratios: 0, 2,000/1, 1,000/1, 800/1, 600/1, 400/1, 200/1. The reaction incubation buffer is 20 mM Tris–HCl pH8, 150 mM NaCl. These samples are incubated at room temperature for 90 min. Thereafter, SDS loading buffer was added to the sample and the mixtures were boiled at 95 °C for 10 min to terminate the proteolytic reaction. At last, the result was detected with SDS–PAGE. Analytical SEC Oligomerization state of His-FL-yTSC1 was analyzed out with Superose 6 Hiload 10/300 GL. Yeast TSC1 fragments, such as wild-type, mutant and truncated forms of yTSC1-CD, as well as hTSC1(1–266), were analysed using a Superdex 200 Hiload 10/300 GL column. Molecular markers (GE Healthcare) of the molecular weights of 669, 440, 158, 75, 44 and 29 kDa represent proteins thyroglobulin, ferritin, aldolase, conalbumin, ovalbumin and carbonic anhydrase, respectively. Human TSC1-NTD homology modelling The structure of hTSC1(1–266) was built using the solved structure of yTSC1-CD from S. pombe as the template. At first, the missing loop regions of yTSC1-CD were built by MODELLER [36] and Rosetta loop modelling [44] . The resulting yTSC1-CD structure was used as final template for homology modelling. In yTSC1-CD structure, every residue and its spatial neighbouring residues form a central residue structure unit (CRSU). The multiple sequence alignment of CRSU was used to construct Hide Markov Model (HMM). The hTSC1(1–266) sequence was used as the query sequence and aligned to yTSC1-CD CRSU HMM. Next, ideal alignment between hTSC1 and yTSC1 was parsed by HMM alignment score. The alignment between query and template sequences was used to construct structure of hTSC1 by MODELLER [36] . The structure of hTSC1(1–67) was modified according to its secondary structure. At last, homology structure of hTSC1-NTD was refined and energy minimized by molecular dynamic simulation [37] . Accession codes: The diffraction data and coordinates of S. pombe TSC1 core domain structures in P2 1 and P2 1 2 1 2 space groups have been deposited in the Protein Data Bank under accession codes 4KK1 and 4KK0 , respectively. How to cite this article: Sun, W. et al. Crystal structure of the yeast TSC1 core domain and implications for tuberous sclerosis pathological mutations. Nat. Commun. 4:2135 doi: 10.1038/ncomms3135 (2013).